Zhang-Rice singlets state formed by two-step oxidation for triggering water oxidation underoperandoconditions 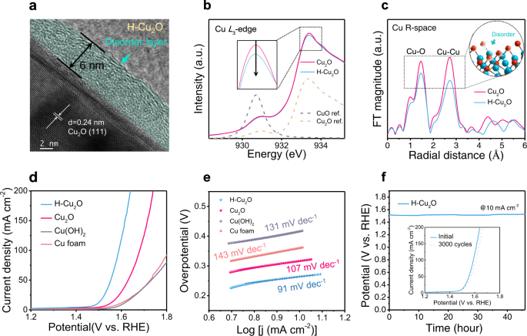Fig. 1: Structural characterization and OER performance of H-Cu2O catalysts. aTEM image of H-Cu2O.bCuL3-edge XANES spectra of Cu2O, H-Cu2O and references (ref.).cCuK-edge EXAFS spectra of Cu2O and H-Cu2O.dOER polarization curves of Cu2O, H-Cu2O, Cu(OH)2, and Cu foam in 1.0 M KOH solution with 90% iR-correction.eThe corresponding Tafel plots of all catalysts.fThe long-term electrochemical stability of H-Cu2O was measured at current density 10 mA cm−2(without iR-correction). The catalyst loadings for Cu2O and H-Cu2O were 11 mg cm−2and 10.8 mg cm−2, respectively. The production of ecologically compatible fuels by electrochemical water splitting is highly desirable for modern industry. The Zhang-Rice singlet is well known for the superconductivity of high-temperature superconductors cuprate, but is rarely known for an electrochemical catalyst. Herein, we observe two steps of surface reconstruction from initial catalytic inactive Cu 1+ in hydrogen treated Cu 2 O to Cu 2+ state and further to catalytic active Zhang-Rice singlet state during the oxygen evolution reaction for water splitting. The hydrogen treated Cu 2 O catalyst exhibits a superior catalytic activity and stability for water splitting and is an efficient rival of other 3 d -transition-metal catalysts. Multiple operando spectroscopies indicate that Zhang-Rice singlet is real active species, since it appears only under oxygen evolution reaction condition. This work provides an insight in developing an electrochemical catalyst from catalytically inactive materials and improves understanding of the mechanism of a Cu-based catalyst for water oxidation. Understanding how the electrocatalyst/electrolyte interface reforms under operating conditions [1] , [2] , [3] , [4] can offer mechanistic insight that allows tracking of the catalytically active motif and enlighten a path towards the development of active and stable electrocatalysts. The nature of such nanoscale interfaces is likely heterogeneous and transforms strongly based on electrochemical operation. To date, however, probing such a dynamic process has been challenging because the surface represents only a tiny fraction of a bulk electrocatalyst, and heterogeneous solid/liquid nanojunctions are nontrivial to characterize in situ [5] , [6] . Electrochemical water splitting for emerging alternative fuels has been considered one of the most feasible tactics to meet the challenge of decarbonization. Identification of the key intermediate state during the oxygen-evolution reaction (OER) [7] , [8] , [9] , which is critical to water splitting and CO 2 reduction reactions, remains elusive. The dynamic evolution of irreversible surface reconstruction on an electrocatalyst during OER and the deciphering of the reaction mechanisms are of utmost importance [6] , [10] , [11] . Engineering the coordination environment of a metal center is of fundamental importance in heterogeneous catalysis [12] , [13] . In particular, modulating the metal–oxygen bonding environment at the electrocatalyst surface offers an effective path toward enhancing the interfacial reactivity. The surface geometric construction and electronic regulation are found to be two decisive factors for the intrinsic improvement of electrocatalytic performance [14] . Accordingly, the first-row 3 d -transition metal (TM) oxides have recently been regarded as promising candidates for OER, owing to their earth abundance and fascinating electronic properties derived from the crystal-field theory. Exemplified by a TM element, the valence variation of a TM plays a pivotal role in catalyzing water oxidation. It is commonly recognized that the high-valent TM species and oxyhydroxides can engender a high reactivity towards OER [15] . Accompanying over-oxidation, the strong hybridization between TM 3 d and O 2 p facilitates the interaction of electrocatalysts and oxygen-related adsorbates [16] , leading to structural disorder and electrochemical irreversibility, which makes tracking technologically challenging. For this reason, it is not straightforward to unravel the nature of the highly covalent bonds in over-oxidized species during OER. Cu-based materials have been proven to be state-of-the-art catalysts for CO 2 reduction [17] , [18] and photocatalytic water reduction [19] . So far the OER performance measured with Cu-based electrocatalysts have, however, fallen far short of a satisfactory standard; in particular, they underperform relative to other late 3 d -TM (e.g., Co and Ni) oxides [20] , [21] . As the cause of this poor performance has not been the focus of extensive studies during the past decade, seeking an inspiring strategy to accelerate OER kinetics on Cu-based electrocatalysts and unveiling their active sites are very challenging but urgent tasks. Herein, the rational regulation of the active Cu center with unsaturated coordination (denoted H-Cu 2 O) via facile hydrogenation is described. Specifically, the substitutional hydrogen induces a surface geometric rearrangement of copper(I) oxide to generate the distinctive oxygen nonstoichiometry, resulting in exceptional performance and durability. Many operando spectroscopic tools, including grazing-angle X-ray scattering (GAXS), quick X-ray absorption (quick-XAS), soft X-ray absorption (soft-XAS), Raman spectra and electrochemical impedance spectroscopy (EIS), were utilized to uncover that the Zhang-Rice singlet state [22] , [23] , [24] , [25] is unexpectedly observed to participate directly in OER-cycle superconductors. For the first time, a Zhang-Rice singlet state is proposed to trigger electrocatalytic oxygen release. Notably, such a high-valent CuO 4 geometry containing Cu 3+ with d 9 L ( L : an O 2 p hole) charged character of Cu d -electrons is a paramount key to dominate the oxygen-evolution step of the OER rather than a CuOOH species, showing a fundamental difference from the conventional scheme. Catalyst characterization A scanning-electron-microscope (SEM) image of the H-Cu 2 O catalyst displays a rod-like morphology (Supplementary Fig. 1 ). This H-Cu 2 O catalyst had disordered surfaces, of which the thickness of the disordered outer layer surrounding a crystalline core was about 6 nm as depicted in illustrated in Fig. 1a . A transmission-electron-microscope (TEM) image and the corresponding fast-Fourier-transform (FFT) patterns of the H-Cu 2 O catalyst further validate the crystalline core covered with a thin structurally disordered layer, induced by the hydrogenation (Supplementary Fig. 2 ). Secondary-ion mass-spectrometry (SIMS) depth profiles of the H-Cu 2 O catalyst illustrate a clear introduction of hydrogen content in the surface of thickness ca. 6–8 nm (Supplementary Fig. 3 ). To understand deeply the disordered surface, multiple techniques, including X-ray photoelectron spectra (XPS) and low-grazing-angle quick-XAS, were employed to characterize the samples as prepared. The Cu 2 p 3/2 XPS spectra show a main feature at ∼ 932.4 eV [26] , corresponding to the chemical state of Cu 1+ or Cu 0 (Supplementary Fig. 4a ). The presence of Cu 1+ for H-Cu 2 O catalyst was confirmed by the dominant signal at 916.8 eV in the Cu LMM spectra (Supplementary Fig. 4b ) [26] . As shown in Fig. 1b , soft-XAS at the Cu- L 3 edge were employed to probe directly the Cu 3 d electronic properties of the H-Cu 2 O catalysts. The main feature at 933.4 eV in Cu 2 O is assigned to the final state 2 p 3/2 p 6 d 10 s 1 from initial state 3 d 10 for Cu 1+ [27] . Clearly, both of Cu 2 O and H-Cu 2 O confirm the presence of Cu 1+ surface. Since Cu 1+ is fully occupied with ten electrons in 3 d , the broad and weak peak at 933.4 is assigned to the unoccupied of 4 s 1 states [27] . Relative to pristine Cu 2 O, the decreased intensity at 933.4 eV indicates that the unoccupied states of 4 s 1 decrease in H-Cu 2 O. This result shows slight charge localization induced by hydrogenation, likely leading to more rapid charge transfer for the OER. X-ray absorption near-edge structure (XANES) and extended X-ray absorption fine structure (EXAFS) were further recorded to reveal the chemical state and local structure of the H-Cu 2 O catalysts. Note that there is no obvious energy shift between Cu 2 O and H-Cu 2 O in the Cu K -edge XANES spectra, exhibiting the primary Cu 1+ features (Supplementary Figs. 5 , 6 ). The result agrees with the Cu LMM Auger spectra (Supplementary Fig. 4b ). The Fourier-transformed k 3 -weighted EXAFS spectra (Fig. 1c) , in which two main features at ~1.5 Å and 2.7 Å correspond to the scattering paths of the nearest oxygen (Cu−O) and the secondary copper atoms (Cu−Cu), testify that most coordination sites of the unsaturated Cu centers appear in the H-Cu 2 O catalysts. Based on these observations, we believe that the H dopant could reform the local electronic configuration and atomic arrangement of bonded Cu and adjacent O atoms and consequently enhance the localization capacity of charges on Cu atoms. In theory, the bonding strength of oxygen intermediates could depend on the degree of the filling in the antibonding states [28] . The enhanced localization capacity of charges on Cu could contribute to much filling of the antibonding states, resulting in weak adsorption of oxygen intermediates. In contrast, the less filling of the antibonding states would result in the strong adsorption of oxygen intermediates. According to OER volcano plot in metal oxides, the binding strength with oxygen intermediates should be neither too strong nor too weak [29] . For p-type Cu 2 O, the highest occupied d -state is quite closer to the Fermi level, resulting in the less filling of antibonding states and the stronger adsorption of oxygen intermediates. Since the adsorption of oxygen on Cu 2 O is too strong that restricts OER activity, the H-Cu 2 O is effective for filling much of the antibonding states with weak intermediates adsorption, and thus achieving a better activity [30] . Fig. 1: Structural characterization and OER performance of H-Cu 2 O catalysts. a TEM image of H-Cu 2 O. b Cu L 3 -edge XANES spectra of Cu 2 O, H-Cu 2 O and references (ref.). c Cu K -edge EXAFS spectra of Cu 2 O and H-Cu 2 O. d OER polarization curves of Cu 2 O, H-Cu 2 O, Cu(OH) 2 , and Cu foam in 1.0 M KOH solution with 90% iR-correction. e The corresponding Tafel plots of all catalysts. f The long-term electrochemical stability of H-Cu 2 O was measured at current density 10 mA cm −2 (without iR-correction). The catalyst loadings for Cu 2 O and H-Cu 2 O were 11 mg cm −2 and 10.8 mg cm −2 , respectively. Full size image Electrochemical properties toward OER activity The OER catalytic performance of the H-Cu 2 O catalysts was evaluated using linear-sweep voltammetry (LSV) in KOH solution (1 M) at scan rate 1 mV s –1 . With a definite coordination-unsaturated structure, the H-Cu 2 O model catalysts exhibit a small overpotential 263 mV, small Tafel slope 91 mV dec –1 and high durability over 45 h at a current density 10 mA cm –2 for OER in alkaline media (Fig. 1d–f ). Such an exceptional performance is superior to those of previously reported 3 d TM-oxide catalysts (Supplementary Fig. 7 ). To well evaluate the stability of H-Cu 2 O, the long-term durability at 10 mA cm –2 and 100 mA cm –2 are tested (Supplementary Figs. 22 , 25 and 28). Evidently, the results show negligible decay of H-Cu 2 O after OER-100 hours of operation with 93% Faradaic efficiency, indicating good stability of the reconstructed surface. Apart from the overpotential and Tafel slope, the electrochemically active surface area (ECSA), which is estimated from the double-layer capacitances ( C dl ), is another significant controlling factor for the intrinsic activity of catalysts. The C dl value of H-Cu 2 O is 13.7% greater than for Cu 2 O, indicating that hydrogenation certainly augments the number of active sites, which is beneficial for the OER (Supplementary Fig. 8c ). To exclude the contribution of larger ECSA for OER performance, a histogram of specific activity of the catalysts with error bar at 1.6 V vs. RHE is given (Supplementary Fig. 8d ), reflecting good intrinsic electrocatalytic activity in H-Cu 2 O catalysts. We conclude that the improved OER performance of the H-Cu 2 O catalysts is attributed to not only the increased ECSA but also the enhanced intrinsic activity owing to the enriched electron densities and coordinatively unsaturated Cu centers. In addition, the H-Cu 2 O catalysts disclose a small resistance of charge transfer relative to Cu 2 O as extracted from EIS analyses (Supplementary Fig. 9 ). To probe the OER kinetics and the properties of the catalyst/electrolyte interfaces, we exploited operando EIS measurements (Supplementary Fig. 10 ). As displayed in the 3D contour Bode plots during OER, the phase-angle relaxation at the low-frequency region (10 0 –10 1 Hz) is closely related to the charge transfer at catalyst/electrolyte interfaces. When the applied potential increase, the phase-angle of H-Cu 2 O at low-frequency region decreases quickly relative to Cu 2 O, indicating the superfast OER kinetics due to the low-coordinated environment of Cu atoms. Identification of the active site To capture the dynamic structural reconstruction or transformation of the catalysts, we implemented operando GAXS and operando quick-XAS during the OER operation. To obtain a more intuitive impression, a customized operando liquid electrochemical cell was designed as depicted in Fig. 2a . 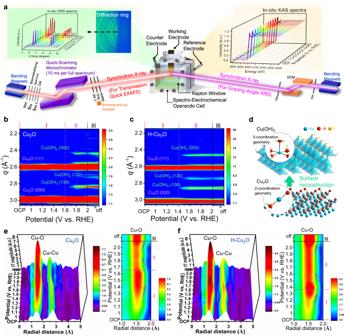Fig. 2:OperandoGAXS and quick-XAS characterizations for the OER. aSchematic illustration of theoperandoliquid electrochemical cell for the GAXS and quick-XAS apparatus.OperandoGAXS of (b) pure Cu2O and (c) H-Cu2O catalysts.dProposed structural reconstruction during OER.OperandoFourier-transformed EXAFS of (e) pure Cu2O and (f) H-Cu2O catalysts (stages I, II and III are assigned to hydroxylation, oxygen evolution and after OER (potential off), respectively). 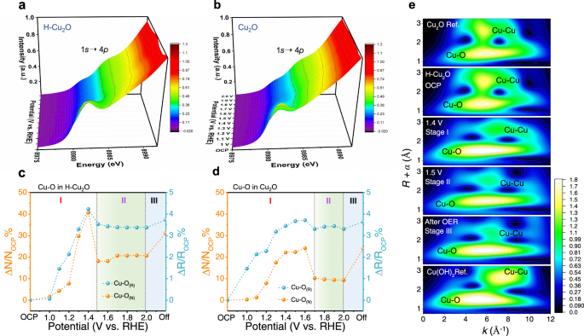Fig. 3: Understanding the correlation between OER activity and local structure transformation. a,b3D patterns ofoperandoCuK-edge XANES of H-Cu2O and Cu2O catalysts.c,dStructural coherence change of Cu–O in EXAFS coordination number (N) and bond length (R) of H-Cu2O and Cu2O catalysts under an applied potential relative to the OCP state.eComparison of CuK-edge WT-EXAFS recorded for H-Cu2O, standard references (Ref.) and catalytic materials at OCP, 1.4, 1.5 V and after OER (stages I, II, and III are assigned to hydroxylation, oxygen evolution and after OER (potential off), respectively). Figure 2b, c presents 2D contour plots of the color-coded scattering intensities as a function of applied potential for the catalysts recorded with operando GAXS at 18 keV of synchrotron X-ray. Stages I, II, and III are assigned to hydroxylation, oxygen evolution and after OER (potential off), respectively. The main characteristic scattering signals are attributed to Cu 2 O (111) and Cu 2 O (200) facets throughout the entire potential range. In region II, the formation of a Cu(OH) 2 phase on the surface of catalysts is captured in both Cu 2 O and H-Cu 2 O catalysts. Such Cu(OH) 2 phases well retain their situation under a potential-off condition, indicating an irreversible surface reformation from Cu 2 O to Cu(OH) 2 (Fig. 2d ). Relative to pure Cu 2 O, stage II at a much smaller potential (below 1.5 V) for H-Cu 2 O catalysts is observed, inferring more rapid deprotonation on the reconstructed surface of Cu 2 O catalysts. Fig. 2: Operando GAXS and quick-XAS characterizations for the OER. a Schematic illustration of the operando liquid electrochemical cell for the GAXS and quick-XAS apparatus. Operando GAXS of ( b ) pure Cu 2 O and ( c ) H-Cu 2 O catalysts. d Proposed structural reconstruction during OER. Operando Fourier-transformed EXAFS of ( e ) pure Cu 2 O and ( f ) H-Cu 2 O catalysts (stages I, II and III are assigned to hydroxylation, oxygen evolution and after OER (potential off), respectively). Full size image Operando Cu K -edge XANES spectra of the H-Cu 2 O catalysts and pristine Cu 2 O under the OER are provided in Supplementary Fig. 11 . The edge energy of H-Cu 2 O at open-circuit potential (OCP) is identical to that of pure Cu 2 O, confirming the nature of Cu 1+ . Upon increasing the anodic potentials, the absorption edge of Cu K -edge XANES spectra for H-Cu 2 O rapidly shifts to greater energies relative to pure Cu 2 O, supporting a more rapid deprotonation on the reconstructed surface of the H-Cu 2 O catalysts [31] , [32] . To probe the electronic structure of the catalysts during OER process, we recorded operando Cu K -edge XANES spectra. The absorption edge (the first-derivative signal) denoted with a dotted line in Fig. 3a, b , shows a smaller energy shift with increased applied voltage, indicating an increased average Cu valence state. A sharp shift was located at a smaller potential (1.4 V) for H-Cu 2 O catalysts vs. 1.6 V for Cu 2 O. Besides, the appearance of a slight shoulder at ∼ 8985 eV on the rising K -edge XAS at applied voltage 1.5 V for H-Cu 2 O and 1.7 V for Cu 2 O, respectively. The feature can be assigned to four-coordinated square–planar geometry [33] . On this basis, the oxidation state of the copper site at stage II might be assigned as +3, showing the electrochemically driven conversion of Cu(OH) 2 into CuO 4 geometry probably. We recorded also the operando Cu K -edge k 3 -weighted EXAFS spectra, which are sensitive to the local crystal structures of an absorbing metal ion. The fitted profiles of Fourier-transformed EXAFS spectra (FT-EXAFS) as results are presented in Supplementary Figs. 12 and 13 and Supplementary Tables 1 and 2 , respectively. As shown in Fig. 2e, f , the corresponding 3D FT patterns along with 2D contour plots reveal a remarkable two-step dynamic structural evolution during electrochemical operation. The detailed coordination environment involving the relative coordination numbers and bond lengths of Cu centers is summarized quantitatively in Fig. 3c and Supplementary Fig. 14 . Before the oxygen evolution (i.e., region I), the coordination numbers (Δ N / N OCP ) and bond lengths (Δ R / R OCP ) of Cu−O for H-Cu 2 O catalysts sharply increased when the applied potential was greater than OCP. For H-Cu 2 O catalysts, the largest Δ N / N OCP and Δ R / R OCP were obtained at the onset of OER at 1.4 V, because of a phase transition from Cu 2 O to Cu(OH) 2 (Fig. 3c ). In contrast, Δ N / N OCP and Δ R / R OCP of pure Cu 2 O slowly increased with applied potential up to 1.6 V (Fig. 3d ). Note that the hydrogenation treatment is an effective route to accelerate Cu pre-oxidation and surface reconstruction during OER. As the applied potential increased further to 1.6 V (i.e., region II), Δ N / N OCP and Δ R / R OCP of the catalysts decreased gradually, likely implying the electrochemical oxidation of Cu(OH) 2 to form an over-oxidized Cu species during oxygen evolution (Supplementary Fig. 14 ). This is also accordant with the operando XANES spectra (Fig. 3a, b ). Such structural reconstruction of Cu species for H-Cu 2 O catalysts is also evident from the wavelet transform (WT) analyses of EXAFS spectra as depicted in Fig. 3e . Two dashed lines at 5.6 and 7.7 Å –1 are defined as the strongest oscillation amplitudes of Cu–O and Cu–Cu bonds. The yellow region represents the FT magnitude of the Cu–O and Cu–Cu bonds in H-Cu 2 O during OER and two references located about 1.8 and 2.7 Å. In the OCP state, the coordination environment of Cu in H-Cu 2 O was confirmed as Cu 2 O because of a similar pattern. On switching on a voltage, a phase transition from H-Cu 2 O toward Cu(OH) 2 occurred (stage I). Fig. 3: Understanding the correlation between OER activity and local structure transformation. a , b 3D patterns of operando Cu K -edge XANES of H-Cu 2 O and Cu 2 O catalysts. c , d Structural coherence change of Cu–O in EXAFS coordination number (N) and bond length (R) of H-Cu 2 O and Cu 2 O catalysts under an applied potential relative to the OCP state. e Comparison of Cu K -edge WT-EXAFS recorded for H-Cu 2 O, standard references (Ref.) and catalytic materials at OCP, 1.4, 1.5 V and after OER (stages I, II, and III are assigned to hydroxylation, oxygen evolution and after OER (potential off), respectively). Full size image Upon further increased applied voltage from 1.4 V, Cu(OH) 2 was further transformed to a operando -generated copper species, which has different patterns for Cu–O and Cu–Cu bonds in stage II. In addition, the Cu–Cu bond shows a different amplitude distribution between stages I and II in the k -space from 7.7 to 6.1 Å –1 . After OER, the pattern of the Cu–Cu bond shifted to a larger k value and a larger Cu–Cu bond distance; phase III was formed. The surface chemistry of H-Cu 2 O catalysts was hence notably altered by dynamic surface reconstruction during OER. This effect indicates that the reconstruction facilitated by hydrogenation is the vital key to evolve oxygen effectively. The electronic structures of the real active sites in H-Cu 2 O catalysts during the OER were well assessed using operando soft-XAS (Fig. 4 ) at the Cu L 3 -edge and O K -edge as known from previous studies on the high-temperature superconductors (high- T c ) Cu superconductors [34] , [35] and even more complicated Cu oxide [36] , [37] . The major challenge is to separate the liquid from the ultrahigh vacuum for OER experiments. 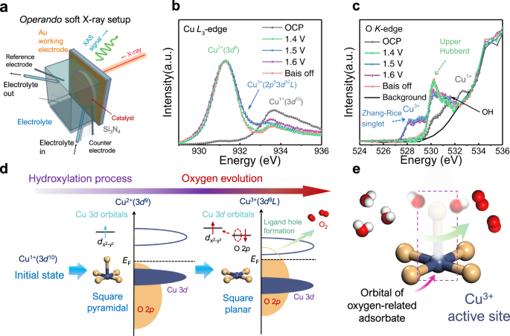Fig. 4:Operandosoft-XAS characterization of high-valent Cu as an active site during OER. aSchematic illustration ofoperandosoft-XAS setup under ultrahigh vacuum condition.bCuL3-edge andcOK-edge of H-Cu2O.dElectronic spin states and orbital physics of Cu site in OER.eSchematic illustration of copper geometry site interaction with oxygen-related adsorbate during oxygen evolution. 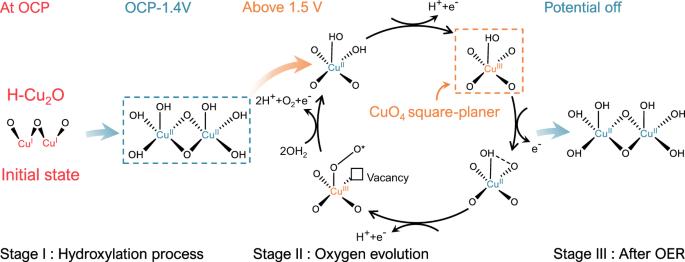Fig. 5: Proposed OER mechanism for H-Cu2O. Dynamic configuration of active sites during OER. Figure 4a shows an operando flow cell with an ultrathin Au@Si 3 N 4 membrane window to separate the liquid cell from the ultrahigh vacuum condition. Figure 4b shows the Cu- L 3 XAS of H-Cu 2 O in regions I–III. At the beginning of stage I (OCP state), we see a broad feature at 933.4 eV (black circles) for an initial Cu 1+ (3 d 10 ) state. A sharp feature at 931.3 eV appeared at applied voltage 1.4 V in region II (green circles) and is assigned to Cu 2+ (2 p 5 3 d 10 final state from 3 d 9 initial state) from Cu(OH) 2 . Most interestingly, a high broad shoulder feature at 932.4 eV appeared under the OER condition, which is well known in the observed La 1–x Sr x CuO 4 (Supplementary Fig. 15 ) corresponding to the doped hole for Cu 3+ state with 2 p 5 3 d 10 L final state [34] , [35] , [38] ( L denotes a hole in the O 2p states). This completely agrees with the operando XANES results (Fig. 3a, b ). The spectral weight of this final state is weak as doped holes are located mainly at the O 2p state [19] , [38] . Upon switching off the applied voltage, this Cu 3+ state immediately vanished and only Cu 2+ remained. As the doped holes are located mainly at the O 2 p states, the quantitative content of the related state Cu 3+ is expected to be observed from the O- K XAS spectra. It is well known that for a charge-transfer system with increased valence state, the pre-edge features shift to lower energy, and their spectral weight increases [35] , [39] . Fig. 4: Operando soft-XAS characterization of high-valent Cu as an active site during OER. a Schematic illustration of operando soft-XAS setup under ultrahigh vacuum condition. b Cu L 3 -edge and c O K -edge of H-Cu 2 O. d Electronic spin states and orbital physics of Cu site in OER. e Schematic illustration of copper geometry site interaction with oxygen-related adsorbate during oxygen evolution. Full size image As shown in Fig. 4c , a strong pre-edge peak at 530.3 eV occurs under an applied voltage below 1.4 V, which is assigned to the transitions to the upper Hubbard band from the O 1 s core level (corresponding to the Cu 2+ state for simplicity). Under OER conditions (stage II) a feature below 529 eV was observed, which is attributable to transitions from O1 s to the doped hole states constructed by the strong O 2 p -Cu 3 d hybridization so-called Zhang-Rice singlet state or Cu 3+ state [35] . A similar feature was recently observed also for cuprate superconductor Ba 2 CuO 4–y , wherein the local octahedron is in an exceptionally compressed version [40] . Both the Cu- L 3 and the O- K XAS spectra hence demonstrate the existence of a Zhang-Rice singlet state or Cu 3+ state under OER conditions. The Cu 3+ (3 d 9 L ) states are split into two poorly resolved peaks at 528.17 eV and 529 eV. A similar splitting was observed in Sr 14 Cu 24 O 41 originating from a different local environment of oxygen ions [36] , [41] (Supplementary Fig. 16c ). Note that the Zhang-Rice singlet state disappeared upon switching off the applied voltage, which means that this real OER active species cannot be observed in experiments ex situ. In addition to the Cu 3+ species, a feature at 531.4 eV appears, which can be assigned to a CuO x (OH) y -related intermediate [1] . After switching off the applied voltage, those features disappear. To obtain the detailed spectral weight of the Zhang-Rice singlet-state-related spectral weight under OER conditions, we analyzed the O- K XAS (black circles) after subtracting an edge jump (black line in Fig. 4c ) in the same way as used for high- T c Cu superconductors [34] as shown in Supplementary Figs. 16a and 17 with the O- K XAS of La 2–x Sr x CuO 4 [34] (Supplementary Fig. 16b ) for comparison. The relative spectral weight of Cu 3+ species corresponds to x = 0.1 in La 2– x Sr x CuO 4 . Proposed catalytic mechanism Based on all above operando X-ray spectroscopic data, a schematic electronic structure at 1.4 V and under OER conditions is depicted in Fig. 4d . As a first step, Cu 2 O with Cu 1+ (3 d 10 ) state transfers gradually to Cu(OH) 2 below 1.5 V in the region I. The Cu 2+ ion in the Cu(OH) 2 phase has a five-coordinated square-pyramidal geometry. On further increasing the applied voltage, part of Cu 2+ was transferred to Cu 3+ (3 d 9 L ) in CuO 4 with four-coordinated square–planar geometry in stage II. After switching off the applied voltage, the Cu 3+ (3 d 9 L ) species returned to the Cu(OH) 2 state. With the valence state of the late TM ion increased by one unit, the charge transfer energy decreased by 3–4 eV and even became a negative value. The O 2 p character gained weight above E F and shifted near E F [42] , [43] , which means that the covalence between Cu 3 d and O 2 p increased from Cu 1+ to Cu 2+ and further to a Cu 3+ state. Previous work indicated that the catalytic activity of TM oxides could be enhanced on increasing the covalence between TM 3 d and oxygen 2 p orbitals [6] . Figure 4e shows the oxygen generation from the surface of H-Cu 2 O at the Cu 3+ (3 d 9 L ) state, which had a square–planar geometry with a bare Cu 3+ as an active site. The CV analyses for catalysts at scan rate of 5 mV s –1 are supplemented to support the in situ generation of Cu 3+ species as shown in Supplementary Fig. 26 . During the oxidation process, only one anodic peak appeared at low potential and was attributed to the conversion of Cu(I) into Cu(II). Coincidentally, the anodic peak of Cu(II)/Cu(III) oxidation at the high- potential region highly overlapped the large OER current response. Even so, in the subsequent reduction process on the reverse potential scan, the broad cathodic peak was observed and resulted from the reductive transformation of Cu(III) to Cu(II). To explore further the unique geometry sites, we recorded operando Raman spectra of H-Cu 2 O in KOH (1.0 M). The Raman spectra in Supplementary Fig. 18 show a comparison of H-Cu 2 O and references. As shown in Supplementary Fig. 19a , the spectra also exhibited two major parts, stage I (hydroxylation below 1.5 V) and II (oxygen evolution above 1.5 V). The H-Cu 2 O phase transition was gradual from Cu 2 O to Cu(OH) 2 with increasing potential in stage I. Three peaks appeared at 292.2, 490.1, and 3557.4 cm –1 , of which the latter corresponds well to the stretching vibration of O–H in Cu(OH) 2 reference. In stage II, a peak at 603.9 cm –1 appeared, due mainly to the framework vibration of Cu–O in CuO 4 [44] . In the deuterium water experiment (Supplementary Fig. 19b ), the peak at 490.1 cm –1 obviously shifted to 480.1 cm –1 with a shift ratio of 97.9%, which further proves that the 480.1 cm –1 peak is attributed to the Cu–OH structure. Furthermore, the redshift of 3557.4 cm –1 to 2628.8 cm –1 verifies the existence of the O–H structure. It must be clarified that there is no obvious redshift at 605.1 cm –1 in the deuterium experiment, indicating that there is no H in this structure. In addition, the potential is also relevant to the appearance and disappearance at of the peak at 605 cm –1 (Supplementary Fig. 20 ). The structure CuO 4 disappeared quickly when the potential was cut off. It demonstrates that CuO 4 is the active structure; this result is consistent with previous X-ray measurements. A continuous phase transition can also be demonstrated in the TEM images of H-Cu 2 O catalyst as shown in (Supplementary Fig. 21 ). After the OER catalytic process, the H-Cu 2 O crystal structure consisted of a Cu 2 O core (circle I) and a Cu(OH) 2 shell (circle II) (Supplementary Fig. 21a ). The crystal planes related to the Cu 2 O core and Cu(OH) 2 shell were also identified in SAED patterns, which is consistent with previous GAXS patterns (Supplementary Fig. 21b, c ). The average depth (~30 nm) of the surface layer of outer Cu(OH) 2 was further observed on an enlarged scale of TEM images (Supplementary Fig. 21d–f ), but the reaction depth (~30 nm) is much larger than a disorder layer (~6 nm) as such reconstruction occurred also for a pure Cu 2 O phase. Another interesting finding is the further generation of an amorphous region on the catalyst surface. The amorphous region has putative active sites that are tuned back from the oxygen-related species during the OER. These operando X-ray measurements and TEM results indicate that the structural disorder led to the rapid surface reconstruction at H-Cu 2 O in OER [31] , [45] . Taking into account all complementary information from multiple operando experiments including GAXS, quick-XAS, soft-XAS, Raman, and EIS, the active-site configuration and reaction cycle are proposed in Fig. 5 , taking advantage of the fact that OH − is preferentially adsorbed on the region of the coordinative unsaturation, and additionally the intrinsic tendency of O 2 p to favor the delocalization of local electrons for a noticeable transformation of the pre-designed metal–oxygen bonding environment. The impact of the hydrogenation on H-Cu 2 O is observed herein to generate the coordinatively unsaturated Cu centers with strong charge localization, which allows the Cu cations to be easily over-oxidized, thereby leading to a facile transformation to high-valent CuO 4 geometry [44] . It is noticeable that we report on operando spectroscopic observations of the Zhang-Rice singlet state responsible for managing the oxygen-evolution step in the form of high-valent Cu 3+ with d 9 L configurations as revealed by soft-XAS. To the best of our knowledge, a Zhang-Rice singlet state serving as active center has not yet been observed for OER electrocatalysts to date. Our results provide direct evidence of high-valent CuO 4 sites, rather than oxyhydroxide species, as the key intermediate state of the pre-equilibrium step on H-Cu 2 O for oxygen evolution. Furthermore, as shown in Supplementary Fig. S23 , the H-Cu 2 O catalyst exhibits pH-dependent OER activity, implying that non-concerted proton-electron transfers may participate in catalyzing the OER [46] . Under alkaline conditions, electrochemically driven deprotonation results in the intramolecular hydroxyl nucleophilic attack pathway where the adjacent OH − attacks CuO 4 to form the O–O bond. Therefore, a pH-dependent nucleophilic attack pathway for O–O bond formation might be presented as shown in Supplementary Fig. S24 . Fig. 5: Proposed OER mechanism for H-Cu 2 O. Dynamic configuration of active sites during OER. Full size image As demonstrated for H-Cu 2 O electrocatalysts, several operando spectral methods allowed us to disentangle the dynamic restructuring during OER at nanoscopic solid/liquid interfaces. This report is the first of the unexpected observation of the Zhang-Rice physics responsible for managing the oxygen-evolution step in the form of high-valent Cu 3+ with d 9 L charge character. Specifically, maximizing the hybridization between Cu(3 d ) and O(2 p ) states with the additional appearance of a ligand hole in O 2 p orbitals favors oxygen-evolution catalysis involved in the OER cycle. Notably, the nature of the definite Zhang-Rice singlet state corroborates the high-valent CuO 4 geometry with four-coordinated square–planar geometry that served as the key intermediate state in the pre-equilibrium step. As far as we are aware, this unusual observation is in sharp contrast with the commonly proposed scheme, predicting an oxyhydroxide species as the active center for OER electrocatalysts. Our work emphasizes that the charge and spin states of TM oxides would be essential to catalyze oxygen evolution during water oxidation. Preparation of pristine Cu 2 O and H-Cu 2 O electrodes The electrodeposition of Cu 2 O was implemented in a two-electrode configuration, including working (Cu foam) and counter (platinum foil) electrodes. The Cu foam was cleaned with sequential ultrasonic treatments in hydrochloric acid (1 M) and deionized water for 10 min each. The surficial Cu(OH) 2 layer on the Cu foam was formed by the subsequent anodization in a NaOH solution (1 M). The electrodeposition condition was performed under a constant current density 4.5 mA cm –2 at 18 °C until the potential 1.6 V was reached. These Cu 2 O electrodes with surficial Cu(OH) 2 layers were rinsed with copious water, dried in air and annealed at 500 °C (heating rate 5 °C min –1 ) in a tubular furnace with a flowing nitrogen stream for 5 h. Preparation of H-Cu 2 O electrodes In a typical synthetic procedure of a hydrogenation treatment, the H-Cu 2 O electrode was set up based on pristine Cu 2 O on applying gaseous H 2 (99.999%) as the hydrogen source. First, the pristine Cu 2 O electrode was placed in a tubular silica furnace and kept under vacuum for 1 h. The furnace was then filled with hydrogen near room temperature. After annealing at 100 °C for 36 h under 1.5 bar H 2 atmosphere we obtained H-Cu 2 O electrodes. The catalyst loadings for Cu 2 O and H-Cu 2 O were 11 mg cm −2 and 10.8 mg cm −2 , respectively. Characterization The morphology of the catalysts was characterized using SEM (JEOL, JSM-6700F) and TEM (JEOL, ARM-200FTH). The high-resolution XPS were measured at TLS beamline BL-24A of the National Synchrotron Radiation Research Center (NSRRC), Taiwan. The XPS measurements were performed under ultrahigh vacuum condition (<10 –6 bar). The binding energies of collected spectra were calibrated to Au 4 f 7/2 of 84 eV for comparison. The XANES measurements were performed at Taiwan beamline BL-12XU in Spring-8, Japan. Athena software was used to process the acquired EXAFS data. The soft-XAS was collected in fluorescence mode at TLS beamline BL-11A of NSRRC, Taiwan. Electrochemical measurements All electrochemical measurements were made out at room temperature in a typical three-electrode system with an electrochemical potentiostat (CHI 6278E, CHI Instruments). The counter and reference electrodes were platinum foil and Hg/HgO, respectively. All applied potentials were calibrated to a reversible hydrogen electrode (RHE, E RHE ) for comparison, as shown in Equation. (1) E RHE = E Ref + 0.059 pH + E Exp . ( E RHE (V): the potential of reversible hydrogen electrode; E Ref (V): the potential of reference electrode; E Exp (V): the potential of working electrode). For OER measurements, cathodic linear-sweep voltammetry with scan rate 1 mV s −1 was performed in KOH (1.0 M, pH ~13.6). The 90% iR compensation was applied for OER test by using the automated iR-correction function of the potentiostat. Gas chromatography (GC) was used to determine the Faradaic efficiency. The ECSA was estimated from the electrochemical double layers of the catalyst surface using Equations. (2) C dl = i v /(dE/dt) and (3) ECSA = C dl / C S . (where C dl is the double-layer capacitance and dE/dt is the scan rate.) The potential windows were measured from 1.1 to 1.2 V versus RHE. The geometric areas of the electrodes were calculated on dividing the general specific capacitances of C s = 40 µF cm −2 for TM oxide in alkaline solution [47] . Operando EIS measurements The EIS were performed in a frequency range from 10 −1 to 10 4 Hz with a small AC amplitude, 10 mV, under applied potential range from 1 to 2 V versus RHE. Operando GAXS measurements The GAXS was performed at beamline BL12-B2 of SPring-8 in Hyogo, Japan. The GAXS patterns were collected with a large Debye–Scherrer camera. The scattering angle was aligned to the Bragg peak of standard CeO 2 powder (SRM 674b). The incident grazing angle of the X-ray was set at 1°; the X-ray energy was 15 keV ( λ = 0.82656 Å). Operando GAXS measurements were performed in a self-assembled Teflon cell sealed with a Kapton tape window (2 × 2 cm 2 ) that was similar to the three-electrode electrochemical condition. The applied potential on the electrode was measured from 1.0 to 2.0 V versus RHE with CHI Instruments. The incident X-ray beam was transmitted through the Kapton window and the electrolyte to collect the surficial GAXS pattern of the electrode. Operando quick-XAS measurements The Cu K -edge XAS were measured at the TPS beamline BL-44A in NSRRC, Taiwan. Operando quick-XAS measurements were performed in the aforementioned self-assembled Teflon cell. The X-ray beam was transmitted through the Kapton tape and electrolyte and reached the detector for XAS collection in the transmission mode. Operando soft-XAS measurements The Cu L 3 -edge XAS measurements were performed at the photoemission end-station at beamline BL-11A in NSRRC, Taiwan. Operando soft-XAS were also recorded in a three-electrode setup with the previous self-assembled cell. A gold-covered Si 3 N 4 window was in contact with copper wires as the working electrode; Hg/HgO and platinum wires were respectively used as reference and counter electrodes. The catalyst powders were dispersed in ethanol with Nafion solution (20 μL, 5%, Sigma-Aldrich), and then sonicated for 10 min. The catalyst ink was drop-cast onto the gold-covered Si 3 N 4 window. The X-ray beam was transmitted through the Si 3 N 4 window and reached the detector for soft-XAS spectra collection in the fluorescence mode.